ABL1 regulates spindle orientation in adherent cells and mammalian skin Despite the growing evidence for the regulated spindle orientation in mammals, a systematic approach for identifying the responsible genes in mammalian cells has not been established. Here we perform a kinase-targeting RNAi screen in HeLa cells and identify ABL1 as a novel regulator of spindle orientation. Knockdown of ABL1 causes the cortical accumulation of Leu-Gly-Asn repeat-enriched-protein (LGN), an evolutionarily conserved regulator of spindle orientation. This results in the LGN-dependent spindle rotation and spindle misorientation. In vivo inactivation of ABL1 by a pharmacological inhibitor or by ablation of the abl1 gene causes spindle misorientation and LGN mislocalization in mouse epidermis. Furthermore, ABL1 directly phosphorylates NuMA, a binding partner of LGN, on tyrosine 1774. This phosphorylation maintains the cortical localization of NuMA during metaphase, and ensures the LGN/NuMA-dependent spindle orientation control. This study provides a novel approach to identify genes regulating spindle orientation in mammals and uncovers new signalling pathways for this mechanism. Spindle orientation is essential for morphogenesis, asymmetric cell division and stem cell self-renewal [1] , [2] . There is increasing evidence for the implication of spindle misorientation in mammalian diseases, including tumourigenesis [3] , [4] and polycystic kidneys [5] . Although the molecular mechanisms for spindle orientation are well studied in the invertebrates [1] , [2] , the mechanisms in mammals remain largely unknown. The reasons for this include the lack of established approaches in mammalian cells to survey the molecules required for the spindle orientation. We have previously shown that in non-polarized mammalian adherent cells, such as HeLa cells, spindles are aligned along the cell-substrate adhesion plane, which ensures both daughter cells attached to the substrate after cell division [6] . This spindle orientation depends on integrin-mediated cell-substrate adhesion and requires actin cytoskeleton, astral microtubules, EB1, myosin X and phosphatidylinositol 3,4,5-triphosphate (PtdIns(3,4,5)P3) [6] , [7] . PtdIns(3,4,5)P3 is accumulated in the midcortex during metaphase and recruits the p150 Glued subunit of dynactin/dynein complex to the midcortex, which results in the spindle orientation parallel to the substratum [7] . We have further shown that Cdc42, a Rho family of small GTPase, regulates spindle orientation through two distinct pathways; the Cdc42–PAK2–βPix–actin pathway and the Cdc42–PI3K–PtdIns(3,4,5)P3 pathway [8] . These mechanisms for spindle orientation function not only in HeLa cells but also in nontransformed MCF-10A cells [6] , [7] , [8] . In addition, recent studies have identified several molecules that regulate spindle orientation in both HeLa cells and mouse embryonic tissues [9] , [10] , [11] . Therefore, the simple approach to analyse spindle orientation in HeLa cells may allow us to identify novel regulators for this mechanism in mammals by means of high-throughput screens. The identified molecules could then be analysed in mouse tissues to examine their in vivo requirement for spindle orientation. Here we performed a genome-scale RNA-mediated interference screen of human kinases by using the HeLa cell system and identified ABL1 tyrosine kinase as a novel regulator for spindle orientation. We find that ABL1 regulates spindle orientation not only in HeLa cells but also in mouse epidermis in vivo . Furthermore, we describe that ABL1 regulates spindle orientation through Leu-Gly-Asn repeat-enriched-protein (LGN) and NuMA, the evolutionarily conserved regulatory complexes for spindle orientation. An RNAi screen of kinases required for spindle orientation We have utilized a simple approach for analysing spindle orientation in HeLa cells, in which the spindles are oriented parallel to the cell-substrate adhesion plane [6] . We used a commercially available small interfering RNA (siRNA) library, which targets 719 genes of human kinases and kinase-related molecules with three individual siRNAs per gene. After transfection of the siRNA library in mitotic synchronized HeLa cells, cells were fixed and stained to visualize the spindles. We performed a two-step screening ( Supplementary Fig. S1 ). In the first screening, the spindle orientation in each metaphase cell was blindly scored on a three-point scale by an observer ( n >30 per sample). The distributions of the score were analysed by the Mann–Whitney U -test. The three individual siRNAs per gene were tested. We judged a gene as a hit when it met the following two criteria. First, when the P -values were less than 2.3×10 −5 , a corrected significant level of 0.05 by Bonferroni procedure, in more than two kinds of siRNAs and second, when P -values were less than 1.0×10 −13 in more than one kind of siRNA. We identified 31 genes as the hits ( Supplementary Table S1 , first screening). In the second screening of the 28 candidate genes identified, the spindle angle between the axis of the spindle and that of substratum was calculated using a custom-made ImageJ plugin, which automatically calculates the spindle angle from a series of Z-stack images ( Supplementary Fig. S2 ). The two individual siRNAs per gene were tested. The distributions of the spindle orientation were analysed by the Mann–Whitney U -test ( Supplementary Table S1 , second screening). The statistical results with a corrected significant level of 0.05 by Bonferroni procedure demonstrated that ABL1 was a strong candidate for the regulator of spindle orientation in HeLa cells ( Supplementary Fig. S1 ). ABL1 regulates spindle orientation in HeLa cells In metaphase, spindles were properly oriented parallel to the substratum in the control luciferase siRNA transfected cells but misoriented significantly in the cells depleted with ABL1 by either of the two kinds of siRNAs ( Fig. 1a–c ). The stable expression of mouse ABL1, which is resistant to the human ABL1 siRNA, restored the proper spindle orientation in the ABL1-depleted cells, excluding the possible off-target effects of the used siRNAs ( Supplementary Fig. S3 ). Green fluorescent protein (GFP) tagged-ABL1-wild type (wt), but not kinase-defective (kd) form of ABL1 (GFP-ABL1-kd) or GFP alone, restored the proper spindle orientation in the ABL1-depleted cells ( Fig. 1d,e ). Then, we treated the cells with imatinib mesylate (Gleevec), a selective inhibitor of ABL1. The endogenous ABL1 kinase activity, which could be monitored by the phosphorylation state of CrkL, was significantly inhibited when the cells were incubated with imatinib for more than 10 h ( Supplementary Fig. S4a ). The imatinib treatment for 30 or 10 h, but not 2 h, induced the misorientation of the spindles in a dose-dependent manner ( Supplementary Fig. S4b–d ). From these results, we conclude that ABL1 regulates spindle orientation in HeLa cells in the kinase activity-dependent manner. 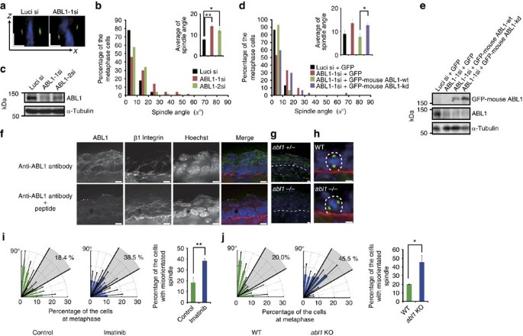Figure 1: ABL1 regulates spindle orientation in HeLa cells and mouse epidermis. (a) Thex–zprojections of metaphase cells transfected with control Luci si or ABL1-1si. (b) Distribution (histogram;n=50) and the average (inset; mean±s.e.m. from three different experiments;n=50 per experiment) of spindle angles in the cells transfected with Luci siRNA or two kinds of ABL1 siRNA (ABL1-1si and ABL1-2 si). *P<0.05 and **P<0.01, analysed by Dunnett's multiple-comparison test. (c) Western blot analysis for ABL1 and control α-tubulin in the cells in (b). (d) Distribution (histogram;n=30) and the average (inset; mean±s.e.m. from four different experiments;n=30 per experiment) of spindle angles in the cells transfected with the indicated siRNAs together with the indicated plasmids. *P<0.05, analysed byt-test. (e) Western blot analysis for GFP-mouse ABL1, endogenous ABL1 and α-tubulin in the cells in (d). (f) Images of E14.5 mouse epidermis which are preincubated with (bottom panels) or without (upper panels) the blocking peptides for anti-ABL1 antibody, and stained with anti-ABL1 (green), anti-β1 integrin antibodies (red) and Hoechst (blue). (g) Images of E16.5 epidermis of ABL1 heterozygous (upper panels) or ABL1 KO (bottom panels) mice stained with anti-ABL1 antibody (green) and Hoechst (blue). The white dotted line indicates the basement membrane. (h) Images of a mitotic cell in E16.5 epidermis from wild-type (WT; upper panels) or ABL1 KO (bottom panels) mice stained with anti-NuMA (green) and anti-β4 integrin (red) antibodies and Hoechst (blue). The white dotted line indicates a cell boundary. (i) Distribution (left; mean±s.d. from three different experiments;n>20 per experiment) and quantification (right; mean±s.d. from three different experiments;n>20 per experiment) of spindle orientation in the control or the imatinib-treated basal cells at E16.5. **P<0.01, analysed byt-test. (j) Distribution (left; mean±s.d. from three different experiments;n=30 per experiment) and quantification (right; mean±s.d. from three different experiments;n=30 per experiment) of spindle orientation in E16.5 basal cells from WT or ABL1 KO mice. *P<0.05, analysed byt-test. Scale bars, 5 μm. Figure 1: ABL1 regulates spindle orientation in HeLa cells and mouse epidermis. ( a ) The x – z projections of metaphase cells transfected with control Luci si or ABL1-1si. ( b ) Distribution (histogram; n =50) and the average (inset; mean±s.e.m. from three different experiments; n =50 per experiment) of spindle angles in the cells transfected with Luci siRNA or two kinds of ABL1 siRNA (ABL1-1si and ABL1-2 si). * P <0.05 and ** P <0.01, analysed by Dunnett's multiple-comparison test. ( c ) Western blot analysis for ABL1 and control α-tubulin in the cells in ( b ). ( d ) Distribution (histogram; n =30) and the average (inset; mean±s.e.m. from four different experiments; n =30 per experiment) of spindle angles in the cells transfected with the indicated siRNAs together with the indicated plasmids. * P <0.05, analysed by t -test. ( e ) Western blot analysis for GFP-mouse ABL1, endogenous ABL1 and α-tubulin in the cells in ( d ). ( f ) Images of E14.5 mouse epidermis which are preincubated with (bottom panels) or without (upper panels) the blocking peptides for anti-ABL1 antibody, and stained with anti-ABL1 (green), anti-β1 integrin antibodies (red) and Hoechst (blue). ( g ) Images of E16.5 epidermis of ABL1 heterozygous (upper panels) or ABL1 KO (bottom panels) mice stained with anti-ABL1 antibody (green) and Hoechst (blue). The white dotted line indicates the basement membrane. ( h ) Images of a mitotic cell in E16.5 epidermis from wild-type (WT; upper panels) or ABL1 KO (bottom panels) mice stained with anti-NuMA (green) and anti-β4 integrin (red) antibodies and Hoechst (blue). The white dotted line indicates a cell boundary. ( i ) Distribution (left; mean±s.d. from three different experiments; n >20 per experiment) and quantification (right; mean±s.d. from three different experiments; n >20 per experiment) of spindle orientation in the control or the imatinib-treated basal cells at E16.5. ** P <0.01, analysed by t -test. ( j ) Distribution (left; mean±s.d. from three different experiments; n =30 per experiment) and quantification (right; mean±s.d. from three different experiments; n =30 per experiment) of spindle orientation in E16.5 basal cells from WT or ABL1 KO mice. * P <0.05, analysed by t -test. Scale bars, 5 μm. Full size image ABL1 regulates spindle orientation in mouse epidermis The skin epidermis is a stratified epithelium, which consists of a single basal layer of proliferative cells that adhere to an underlying basement membrane and the multiple layers of differentiating suprabasal cells [9] , [12] . During development, the basal epidermal cells divide parallel or perpendicularly to the basement membrane, which promotes stratification and two dimensional growth of the epithelium, respectively [9] . Immunostaining with anti-ABL1 antibody showed that at embryonic day 14.5 (E14.5), when most of the epidermis consists of two or three layers of cells, ABL1 was expressed strongly in epidermis but hardly in the underlying dermis ( Fig. 1f,g , upper panels). The signal in epidermis was barely detected when the used antibody was pretreated with blocking peptides or in the ABL1 knockout (KO) epidermis, confirming the expression of ABL1 in epidermis ( Fig. 1f,g , bottom panels). We injected imatinib into the peritoneum of pregnant mice and examined the spindle orientation in the basal epidermal cells of the embryo. Although the spindles ( Fig. 1h ) were properly oriented parallel or perpendicularly to the basement membrane in the control E16.5 epidermis, they were misoriented significantly in the imatinib-treated E16.5 epidermis ( Fig. 1i ). The aberrant spindle orientation was also observed in the imatinib-treated E14.5 epidermis ( Supplementary Fig. S5 ). In addition, spindles were misoriented significantly in the E16.5 epidermis in ABL1 KO mice [13] , [14] , while properly oriented in the wild-type E16.5 epidermis ( Fig. 1h,j ). In the wild-type epidermis, the proportion of the cells with the perpendicular and parallel spindle orientation varies from embryo to embryo, but that with the misoriented spindles is constantly low. In contrast, in the imatinib-treated or ABL1 KO epidermis, the proportion of the cells with the misoriented spindles is significantly increased ( Fig. 1i,j ). Thus, ABL1 regulates spindle orientation not only in HeLa cells but also in mouse epidermis in vivo . ABL1 suppresses the cortical accumulation of LGN How does ABL1 regulate spindle orientation? We have previously shown that PtdIns(3,4,5)P3 and the Pak2–βPix complex are required for the proper spindle orientation in HeLa cells [7] , [8] . However, both the activation of PI(3)K during M phase ( Supplementary Fig. S6a , p-Akt, 9 h) and the complex formation of Pak2 with βPix in M-phase cells ( Supplementary Fig. S6b ) were normal in the ABL1-depleted cells. Then, we investigated the possible involvement of LGN, a mammalian orthologue of Drosophila Pins [1] , [2] , [15] , [16] , [17] , [18] . 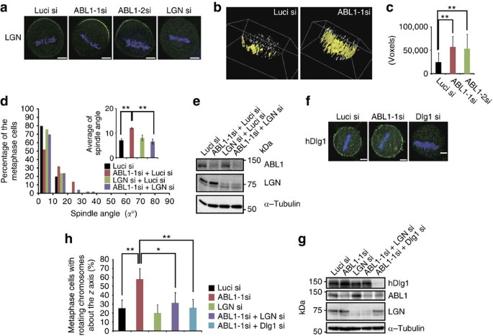Figure 2: ABL1 suppresses the cortical accumulation of LGN to prevent the LGN/Dlg-mediated spindle rotation. (a) Images of metaphase cells transfected with the indicated siRNAs and stained with anti-LGN antibody (green) and Hoechst (blue). (b) The three-dimensionally reconstructed images of metaphase cells transfected with the indicated siRNAs and stained with anti-LGN antibody. The localization of LGN at the cortex is shown in yellow. (c) Quantification of cortical LGN in metaphase cells. The averages (mean±s.d.;n=20) of voxel values for cortical LGN in metaphase cells transfected with the indicated siRNAs are shown. One voxel represents 0.00027 μm3. **P<0.01, analysed by Dunnett's multiple-comparison test. (d) Distribution (histogram;n=40) and the average (mean±s.e.m. from three different experiments;n=40 per experiment) of spindle angles in the cells transfected with the indicated siRNAs. **P<0.01, analysed by Dunnett's multiple-comparison test. (e) Western blot analysis for ABL1, LGN and α-tubulin in the cells in (d). (f) Images of metaphase cells transfected with the indicated siRNAs and stained with anti-Dlg antibody (green) and Hoechst (blue). (g) Western blot analysis for Dlg, ABL1, LGN and α-tubulin in the cells in (h). (h) Quantification of spindle rotation about thezaxis. Values shown are mean±s.d. from three different experiments (n>20 per experiment). *P<0.05 and **P<0.01, analysed by Dunnett's multiple-comparison test. Scale bars, 5 μm. LGN was localized at the cortex in the control metaphase cells ( Fig 2a , luciferase siRNA (Luci si)), which was diminished in the LGN-depleted cells ( Fig 2a , LGN si and Fig. 2e ), confirming the cortical localization of LGN in HeLa cells. Surprisingly, in the ABL1-depleted cells, the cortical signal of LGN was more intense ( Fig. 2a , ABL1 siRNA (ABL1-1si, ABL1-2si)). The three-dimensional reconstruction images of cortical LGN signals show that the depletion of ABL1 broadens the cortical localization of LGN along the z axis ( Fig. 2b ; Supplementary Movie 1 , 2 ). The volumes of the cortical LGN signals were significantly larger in the ABL1-depleted cells than in the control cells ( Fig. 2c ; Supplementary Fig. S7 ), although the total levels of the LGN protein were unchanged ( Fig. 2e ; Supplementary Fig. S6a ). These results demonstrate that ABL1 suppresses the cortical accumulation of LGN during M phase without altering the expression level of the LGN protein in HeLa cells. Figure 2: ABL1 suppresses the cortical accumulation of LGN to prevent the LGN/Dlg-mediated spindle rotation. ( a ) Images of metaphase cells transfected with the indicated siRNAs and stained with anti-LGN antibody (green) and Hoechst (blue). ( b ) The three-dimensionally reconstructed images of metaphase cells transfected with the indicated siRNAs and stained with anti-LGN antibody. The localization of LGN at the cortex is shown in yellow. ( c ) Quantification of cortical LGN in metaphase cells. The averages (mean±s.d. ; n =20) of voxel values for cortical LGN in metaphase cells transfected with the indicated siRNAs are shown. One voxel represents 0.00027 μm 3 . ** P <0.01, analysed by Dunnett's multiple-comparison test. ( d ) Distribution (histogram; n =40) and the average (mean±s.e.m. from three different experiments; n =40 per experiment) of spindle angles in the cells transfected with the indicated siRNAs. ** P <0.01, analysed by Dunnett's multiple-comparison test. ( e ) Western blot analysis for ABL1, LGN and α-tubulin in the cells in ( d ). ( f ) Images of metaphase cells transfected with the indicated siRNAs and stained with anti-Dlg antibody (green) and Hoechst (blue). ( g ) Western blot analysis for Dlg, ABL1, LGN and α-tubulin in the cells in ( h ). ( h ) Quantification of spindle rotation about the z axis. Values shown are mean±s.d. from three different experiments ( n >20 per experiment). * P <0.05 and ** P <0.01, analysed by Dunnett's multiple-comparison test. Scale bars, 5 μm. Full size image ABL1 suppresses the LGN/Dlg-dependent spindle rotation It is reported that the overexpression of LGN causes the spindle-rocking motion in MDCK cells [16] . Consistently, the overexpression of GFP-LGN in metaphase-arrested HeLa cells caused the rotational motion of metaphase chromosomes ( Supplementary Movie 3 ). We hypothesized that the spindle misorientation in the ABL1-depleted cells resulted from the cortical accumulation of LGN, which induced the spindle rotation about the z axis. Supporting this hypothesis, downregulation of LGN restored the proper spindle orientation in the ABL1-depleted cells ( Fig. 2d,e ). In addition, metaphase chromosomes displayed active rotational motions about the z axis in the ABL-depleted cells ( Fig. 2h , ABL1-1si and Supplementary Movie 5 ), but not in the control cells ( Fig. 2h , Luci si and Supplementary Movie 4 ) or in the cells depleted with both ABL1 and LGN ( Fig. 2h , ABL1-1si+LGN si and Supplementary Movie 6 ). These results indicate that, in the ABL1-depleted cells, the spindles are abnormally rotated about the z axis in an LGN-dependent manner. It is noteworthy that the depletion of LGN alone does not induce spindle misorientation or spindle rotational motion about the z axis ( Fig. 2d,e,h ). The inhibition of PI(3)K by LY294002 induces spindle misorientation in the cells depleted with LGN alone or in the cells depleted with both LGN and ABL1 ( Supplementary Fig. S8 ), indicating that the PI(3)K–PtdIns(3,4,5)P3 pathway functions to orient the spindle parallel to the substratum in the absence of LGN. Thus, under normal conditions, ABL1 suppresses the excess accumulation of LGN at the cortex to prevent the abnormal spindle rotation about the z axis induced by the mislocalized LGN. This ensures the PI(3)K–PtdIns(3,4,5)P3 pathway functions normally to orient the spindle parallel to the substratum. In the asymmetric cell division of Drosophila neuroblasts, Pins provides a link between astral microtubules and the cortex through Dlg [19] , [20] . Dlg was localized at the cortex in the control metaphase HeLa cells ( Fig. 2f , Luci si), which was diminished in the Dlg1-depleted cells ( Fig. 2f,g , Dlg1 si), confirming its cortical localization in HeLa cells. In the ABL1-depleted cells, Dlg1 was still localized at the cortex ( Fig. 2f , ABL1-1si). The rotational motions of the metaphase chromosomes in the ABL1-depleted cells were suppressed when the cells were depleted with both ABL1 and Dlg1 ( Fig. 2h , ABL1-1si+Dlg1 si). These results demonstrate that ABL1 suppresses the LGN and Dlg1-dependent spindle rotation about the z axis. ABL1 targets LGN to the apical cortex in epidermis In the wild-type E16.5 basal epidermal cells, LGN was localized to the apical cortex in a crescent shape, as reported previously [9] ( Fig. 3a–c , control and Fig. 3d–g , WT). LGN still formed a crescent in the imatinib-treated or the ABL1 KO E16.5 epidermis, but it was no longer restricted to the apical domain ( Fig. 3a–c , imatinib and Fig. 3d–g , abl1 KO). Sometimes it was localized even in the basal cortex ( Fig. 3d , abl 1 KO) or formed two crescents in a cell ( Fig. 3a , imatinib, arrow). The percentages of the metaphase cells with two LGN crescents were 7% and 32.7% in the WT ( n =57) and the imatinib-treated ( n =55) epidermis, respectively. Thus, ABL1 ensures the apical localization of LGN in mouse epidermis in vivo . Interestingly, in some populations of the laterally dividing cells in the wild-type epidermis, spindles were oriented orthogonal to the apical LGN polarity ( Fig. 3d , WT; Fig. 3e , WT, bottom panel; Fig. 3h , WT), whereas in the ABL1 KO epidermis the populations of the spindles uncoupled with LGN polarity was significantly reduced ( Fig. 3h , abl1 KO). We speculate that, in the WT epidermis, LGN and the lateral cortical cues, including adherens junction proteins, generate a strong pulling force at the apical cortex and a weak pulling force at the lateral cortex, respectively. In the ABL1 KO epidermis, however, LGN randomly positions at the cortex, which induces the imbalance between the pulling forces generated by LGN and that by the lateral cortical cues. This imbalance results in a torque on the spindle, which aligns it along the strong pulling force generated by LGN. 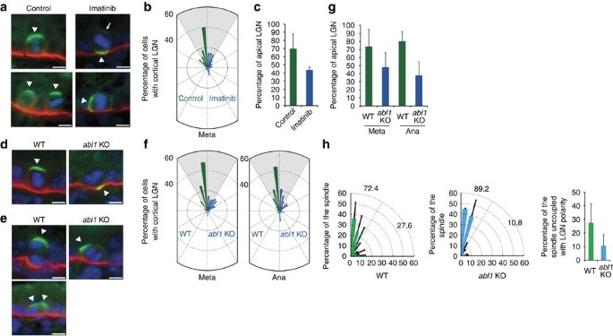Figure 3: ABL1 is required for the apical localization of LGN in mouse epidermis. (a) Images of E16.5 epidermal basal cells in the control or the imatinib-treated embryos stained with anti-LGN (green), anti-β4 integrin (red) antibodies and Hoechst (blue). The arrowhead indicates the LGN crescent at the cortex. The arrow indicates an additional LGN crescent in an imatinib-treated basal cell. (b) Distribution (n>20 per experiment) of the LGN localization at the cortex in the E16.5 control or the imatinib-treated basal cells. LGN localization was determined by the centre of an LGN crescent in a mitotic cell. (c) Quantification of apical LGN (mean±s.d. from two different experiments;n>20 per experiment) in the E16.5 control or the imatinib-treated basal cells. (d,e) Images of E16.5 epidermal basal cells during metaphase (d) or anaphase (e) in the WT or the ABL1 KO mice stained with anti-LGN (green), anti-β4 integrin (red) antibodies and Hoechst (blue). (f) Distribution of LGN localization at the cortex during metaphase (left) or anaphase (right) in the E16.5 WT or the ABL1 KO basal cells (n>20 per experiment). (g) Quantification of apical LGN during metaphase or anaphase (mean±s.d. from two different experiments;n>20 per experiment) in the E16.5 WT or the ABL1 KO basal cells. (h) Quantification of spindle orientation relative to the axis of LGN polarity in the E16.5 WT or the ABL1 KO basal cells in metaphase. Scale bars, 5 μm. Figure 3: ABL1 is required for the apical localization of LGN in mouse epidermis. ( a ) Images of E16.5 epidermal basal cells in the control or the imatinib-treated embryos stained with anti-LGN (green), anti-β4 integrin (red) antibodies and Hoechst (blue). The arrowhead indicates the LGN crescent at the cortex. The arrow indicates an additional LGN crescent in an imatinib-treated basal cell. ( b ) Distribution ( n >20 per experiment) of the LGN localization at the cortex in the E16.5 control or the imatinib-treated basal cells. LGN localization was determined by the centre of an LGN crescent in a mitotic cell. ( c ) Quantification of apical LGN (mean±s.d. from two different experiments; n >20 per experiment) in the E16.5 control or the imatinib-treated basal cells. ( d,e ) Images of E16.5 epidermal basal cells during metaphase ( d ) or anaphase ( e ) in the WT or the ABL1 KO mice stained with anti-LGN (green), anti-β4 integrin (red) antibodies and Hoechst (blue). ( f ) Distribution of LGN localization at the cortex during metaphase (left) or anaphase (right) in the E16.5 WT or the ABL1 KO basal cells ( n >20 per experiment). ( g ) Quantification of apical LGN during metaphase or anaphase (mean±s.d. from two different experiments; n >20 per experiment) in the E16.5 WT or the ABL1 KO basal cells. ( h ) Quantification of spindle orientation relative to the axis of LGN polarity in the E16.5 WT or the ABL1 KO basal cells in metaphase. Scale bars, 5 μm. Full size image ABL1 maintains NuMA at the cortex in metaphase During M phase, NuMA binds to LGN and induces the conformational switch of LGN to an open state, allowing it to associate with Gα at the cortex [16] . NuMA is a microtubule-binding protein and associates with dynein [21] . It is believed that NuMA associates with astral microtubules at the cortex and regulates their attachment to dynein or to a cortical attachment factor to orient the spindle [16] . Consistent with previous reports [16] , [22] , [23] , NuMA was localized at the cortex and along spindle microtubules during prometaphase and metaphase in HeLa cells ( Fig. 4a , Luci si). NuMA was colocalized with LGN at the cortex in metaphase cells ( Supplementary Fig. S9 , Luci si). The localization of NuMA at the cortex, but not that along spindle microtubules, was diminished in the cells transfected with LGN siRNA, indicating that NuMA was localized at the cortex in an LGN-dependent manner, as has been reported previously [16] ( Fig. 4a , LGN si and Supplementary Fig. S9 , LGN si). In the ABL1-depleted cells, NuMA was localized at the cortex in prometaphase cells, but unexpectedly it was diminished from the cortex in metaphase cells, although LGN was localized to the cortex ( Fig. 4a , ABL1-1si and Supplementary Fig. S9 , ABL1-1si and ABL1-2si). In addition, NuMA was localized to the apical cortex in the WT E16.5 epidermis ( Fig. 4b , upper panel), but diminished from the cortex in the ABL1 KO E16.5 epidermis ( Fig. 4b , bottom panel). These results demonstrate that ABL1 is required for maintaining the cortical localization of NuMA during metaphase both in HeLa cells and mouse epidermis. 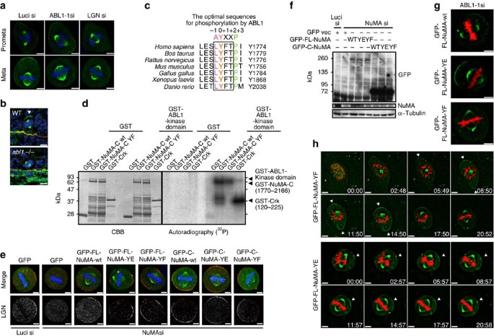Figure 4: ABL1 phosphorylates NuMA on Tyr 1774 and anchors it to the cortex during metaphase. (a) Images of prometaphase (upper panels) and metaphase (bottom panels) cells transfected with the indicated siRNAs and stained with anti-NuMA antibody (green) and Hoechst (blue). (b) Images of E16.5 epidermal basal cells from the WT (upper panels) or the ABL1 KO (bottom panels) mice stained with anti-NuMA (green) and anti-β4 integrin antibodies (red) and Hoechst (blue). The arrowhead indicates the apical localization of NuMA at the cortex. (c) Protein sequence alignment of NuMA from seven vertebrate species, showing a conserved tyrosine residue (Y1774) within an optimal sequence for phosphorylation by ABL1. A: an apolar amino acid; X: any amino acid. (d) Thein vitrokinase assay of GST-ABL1 kinase domain towards the indicated forms of GST-NuMA-C(1770-2166) or GST-Crk(120-225). The images of CBB staining (left) and autoradiography (32P; right) are shown. (e) Images of metaphase cells transfected with the indicated siRNAs together with the indicated forms of GFP-NuMA. The images of LGN (bottom panels) and the merge images (upper panels) of GFP-NuMA (green), LGN (red) and Hoechst (blue) are shown. (f) Western blot analysis for GFP, NuMA and α-tubulin in the cells in (e). (g) Live images of the indicated forms of GFP-FL-NuMA (green) in the ABL1-depleted cells during metaphase. RFP-H2B is shown in red. (h) Time-lapse images of GFP-FL-NuMA-YF (upper panel) or GFP-FL-NuMA-YE (bottom panel) in the ABL1-depleted cells during prometaphase to metaphase. Arrowheads indicate the GFP fluorescence at the cortex. Scale bars, 5 μm. Figure 4: ABL1 phosphorylates NuMA on Tyr 1774 and anchors it to the cortex during metaphase. ( a ) Images of prometaphase (upper panels) and metaphase (bottom panels) cells transfected with the indicated siRNAs and stained with anti-NuMA antibody (green) and Hoechst (blue). ( b ) Images of E16.5 epidermal basal cells from the WT (upper panels) or the ABL1 KO (bottom panels) mice stained with anti-NuMA (green) and anti-β4 integrin antibodies (red) and Hoechst (blue). The arrowhead indicates the apical localization of NuMA at the cortex. ( c ) Protein sequence alignment of NuMA from seven vertebrate species, showing a conserved tyrosine residue (Y1774) within an optimal sequence for phosphorylation by ABL1. A: an apolar amino acid; X: any amino acid. ( d ) The in vitro kinase assay of GST-ABL1 kinase domain towards the indicated forms of GST-NuMA-C(1770-2166) or GST-Crk(120-225). The images of CBB staining (left) and autoradiography ( 32 P; right) are shown. ( e ) Images of metaphase cells transfected with the indicated siRNAs together with the indicated forms of GFP-NuMA. The images of LGN (bottom panels) and the merge images (upper panels) of GFP-NuMA (green), LGN (red) and Hoechst (blue) are shown. ( f ) Western blot analysis for GFP, NuMA and α-tubulin in the cells in ( e ). ( g ) Live images of the indicated forms of GFP-FL-NuMA (green) in the ABL1-depleted cells during metaphase. RFP-H2B is shown in red. ( h ) Time-lapse images of GFP-FL-NuMA-YF (upper panel) or GFP-FL-NuMA-YE (bottom panel) in the ABL1-depleted cells during prometaphase to metaphase. Arrowheads indicate the GFP fluorescence at the cortex. Scale bars, 5 μm. Full size image ABL1 phosphorylates NuMA on Y1774 Recent studies have shown that the Frizzled–Dishevelled planar cell polarity pathway regulates spindle orientation through Mud, the Drosophila NuMA orthologue, and that ABL1 regulates Frizzled–Dishevelled planar cell polarity pathway by phosphorylating Dsh [24] , [25] . In addition, Dvl1, Dvl2 and Dvl3, the mammalian Dsh homologues, have been reported to regulate spindle orientation in HeLa cells [26] . Thus, it might be possible that ABL1 would regulate the cortical localization of NuMA and spindle orientation through Dvl. However, the cortical localization of NuMA and LGN was normal in HeLa cells depleted with all Dvl1, Dvl2 and Dvl3 by RNAi as in the control cells ( Supplementary Fig. S10a–c ). Moreover, the expression of either GFP-Dvl2-wt or GFP-Dvl2-YF, an unphosphorylatable mutant form of Dvl2 in which the ABL1 phosphorylation site Y502 was replaced by phenylalanine, restored the proper spindle orientation in the Dvl2-depleted cells ( Supplementary Fig. S10d and e ). Thus, ABL1 should regulate the cortical localization of NuMA and spindle orientation by a mechanism that is independent of Dvl. Previous phosphoproteomic analyses have shown that Tyr 1774 of NuMA is phosphorylated in the mitotic-arrested HeLa cells [27] , [28] . The amino-acid sequence surrounding Tyr 1774 closely resembles the optimal sequence for phosphorylation by ABL1 (ref. 29 ). Although this sequence is absent from Mud, it is conserved in several vertebrate species ( Fig. 4c ). In addition, the endogenous ABL1 kinase activity was increased in M phase, as reported previously [30] ( Supplementary Fig. S11 ). These findings led us to examine the possibility that ABL1 could directly phosphorylate NuMA on Tyr 1774 and this phosphorylation would ensure the localization of NuMA at the cortex during metaphase. We performed the in vitro kinase assay using recombinant proteins. The GST-fused ABL1-kinase domain significantly phosphorylated the C terminus NuMA (1700–2166; Fig. 4d ), although the efficiency of phosphorylation is slightly lower than that towards Crk, a well-known substrate of ABL1 (ref. 31 ; Fig. 4d , GST-NuMA-C-wt and GST-Crk and Supplementary Fig. S12 ). The phosphorylation was reduced when Tyr 1774 was replaced by phenylalanine ( Fig. 4d , GST-NuMA-C-YF), indicating that ABL1 directly phosphorylates NuMA on Tyr 1774. Y1774 phosphorylation maintains NuMA at the cortex Tyr 1774 lies outside the microtubule and LGN-binding domains in the C terminus NuMA [22] , [32] . Both Myc tagged-full-length (FL) and C terminus (C) NuMA-YF, as well as Myc-FL/C-NuMA-wt and Myc-FL/C-NuMA-YE, in which Tyr 1774 was replaced by glutamic acid to mimic phosphorylation, was co-immunoprecipitated with GFP-LGN ( Supplementary Fig. S13 ). Thus, Tyr 1774 phosphorylation does not alter the binding ability of NuMA towards LGN. LGN is known to be localized at the cortex in a NuMA-dependent manner [16] . Consistently, LGN was not localized to the metaphase cortex in the NuMA-depleted cells ( Fig. 4e , NuMA si, GFP). The expression of the siRNA resistant form of GFP-FL/C-NuMA-wt, -YE or -YF restored the cortical localization of LGN in the NuMA-depleted cells ( Fig. 4e ). In addition, the cortical accumulation of LGN in the ABL1-depleted cells was inhibited by downregulation of NuMA, but restored again by the expression of GFP-FL/C-NuMA-wt, -YE or -YF ( Supplementary Fig. S14 ). The efficiency of the restoration by GFP-FL/C-NuMA-YF was almost the same as that by GFP-FL/C-NuMA-wt and -YE ( Fig. 4e and f ; Supplementary Fig. S14 ). These results demonstrate that the cortical localization of LGN depends on NuMA, but is independent of NuMA-Tyr 1774 phosphorylation. Next, we examined the localization of GFP-FL-NuMA-wt, GFP-FL-NuMA-YF and GFP-FL-NuMA-YE in the ABL1-depleted cells. The live imaging showed that GFP-FL-NuMA-YE, but not GFP-FL-NuMA-wt or GFP-FL-NuMA-YF, was localized to the cortex in the ABL1-depleted metaphase cells, whereas all of them were localized along the spindle microtubules ( Fig. 4g ). Importantly, GFP-FL-NuMA-YF was localized to the cortex during prometaphase, but disappeared from the cortex immediately after the onset of metaphase, whereas GFP-FL-NuMA-YE was persistently localized to the cortex during prometaphase and metaphase ( Fig. 4h ). However, GFP-FL-NuMA-YE was diminished from the cortex in the LGN-depleted cells ( Supplementary Fig. S15a ). Thus, the cortical localization of NuMA requires both LGN and Tyr 1774 phosphorylation. We demonstrate that NuMA is bound to LGN and recruited to the cortex during prometaphase in a LGN-dependent manner and then anchored to the cortex during metaphase in an ABL1-mediated Tyr 1774 phosphorylation-dependent manner. It should be noted that the C-terminal forms of NuMA did not localize at the metaphase cortex ( Supplementary Fig. S15b ), indicating the requirement of the N terminus NuMA for this anchoring mechanism. Y1774 phosphorylation aligns a spindle towards LGN crescent When we closely examined the LGN and spindles in HeLa cells, we realized that LGN formed a crescent at the cortex during metaphase and the spindles were aligned towards the centre of the LGN crescent in metaphase cells ( Fig. 5a–c , Luci si, and Fig. 2a,b ). In the ABL1-depleted cells, LGN still formed a crescent at the cortex, but the spindles were only partially aligned towards the LGN crescent ( Fig. 5a–c , ABL1-1si, and Fig. 2a,b ). Moreover, the expression of GFP-FL-NuMA-YF in the NuMA-depleted cells resulted in the spindle misorientation towards the LGN crescent, whereas it was properly oriented in the cells expressing GFP-FL-NuMA-YE ( Fig. 5d–f ). Importantly, the spindle orientation about the z axis was normal in the NuMA-depleted cells ( Supplementary Fig. 16a ), similar to LGN-depleted cells ( Fig. 2d,e ). In addition, the expression of GFP-FL-NuMA-YF, as well as GFP-FL-NuMA-YE, in the NuMA-depleted cells has no effect on spindle orientation about the z axis ( Supplementary Fig. 16b ). Thus, under normal condition, LGN, NuMA and Y1774 phosphorylation of NuMA regulate spindle orientation towards the LGN crescent on the x – y plane, but have a minor role in regulating spindle orientation about the z axis. In the ABL1-depleted metaphase cells, however, LGN is broadly localized at the cortex along the z axis, which results in the LGN/Dlg-dependent spindle rotation and spindle misorientation, even though NuMA is no longer localized at the cortex ( Figs 2 and 4a,b ). The x – z projection of an ABL1-depleted metaphase cell showed that LGN formed a crescent at the midcortex along the z axis ( Fig. 5g , ABL1-1si+GFP). In these cells, the spindles failed to align towards the LGN crescent in the z axis and thus were tilted. The expression of GFP-FL-NuMA-YE, but not GFP-FL-NuMA-YF in the ABL1-depleted cells, restored the proper spindle orientation towards the LGN crescent in the z axis and as a result, the spindles were oriented parallel to the substratum ( Fig. 5g ). Consistently, the expression of GFP-FL-NuMA-YE, but not GFP-FL-NuMA-wt, restored the proper spindle orientation parallel to the substratum in the ABL1-depleted cells ( Fig. 5h ). These results demonstrate that NuMA-Y1774 phosphorylation maintains the cortical localization of NuMA during metaphase and provides a mechanism to align the spindle towards the LGN crescent, and thus is essential for the LGN/NuMA-dependent spindle orientation control. 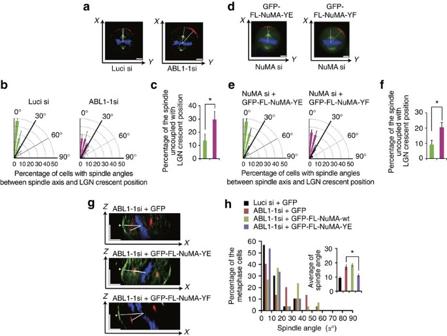Figure 5: Tyr 1774 phosphorylation of NuMA is required for the alignment of the spindle > towards the LGN crescent. (a) Typical images of metaphase cells on thex–yplane transfected with control Luci si or ABL1-1si and stained with anti-LGN (red) and anti-γ-tubulin (green) antibodies and Hoechst (blue). (b) Distribution of spindle angle relative to the centre of the cortical LGN crescent (mean±s.d. from three different experiments;n>30 per experiment). Spindle angles were measured between the white lines in (a). (c) Quantification of spindle misorientation towards the centre of the cortical LGN crescent (populations between 30° and 90° degrees in (b). (d) Images of metaphase cells transfected with NuMA siRNA together with GFP-FL-NuMA-YE (left, green) or GFP-FL-NuMA-YF (right, green) and stained with anti-LGN antibody (red) and Hoechst (blue). (e) Distribution of spindle angle relative to the centre of the cortical LGN crescent (mean±s.d. from three different experiments;n>30 per experiment). Spindle angles were measured between the white lines in (d). (f) Quantification of spindle misorientation towards the centre of the cortical LGN crescent (populations between 30° and 90° degrees in (e). (g) Thex–zprojections of metaphase cells transfected with ABL1 siRNA together with GFP alone, GFP-FL-NuMA-YE or GFP-FL-NuMA-YF, and stained with anti-LGN and anti-γ-tubulin antibodies and Hoechst (blue). The signals for LGN and γ-tubulin are shown in green and red, respectively. GFP signals are not shown. (h) Distribution (histogram;n=30) and the average (inset; mean±s.e.m. from four different experiments;n=30 per experiment) of spindle angles about thezaxis in the cells transfected with the indicated siRNAs together with the indicated plasmids. *P<0.05, analysed byt-test (right). Scale bars, 5 μm. Figure 5: Tyr 1774 phosphorylation of NuMA is required for the alignment of the spindle > towards the LGN crescent. ( a ) Typical images of metaphase cells on the x – y plane transfected with control Luci si or ABL1-1si and stained with anti-LGN (red) and anti-γ-tubulin (green) antibodies and Hoechst (blue). ( b ) Distribution of spindle angle relative to the centre of the cortical LGN crescent (mean±s.d. from three different experiments; n >30 per experiment). Spindle angles were measured between the white lines in ( a ). ( c ) Quantification of spindle misorientation towards the centre of the cortical LGN crescent (populations between 30° and 90° degrees in ( b ). ( d ) Images of metaphase cells transfected with NuMA siRNA together with GFP-FL-NuMA-YE (left, green) or GFP-FL-NuMA-YF (right, green) and stained with anti-LGN antibody (red) and Hoechst (blue). ( e ) Distribution of spindle angle relative to the centre of the cortical LGN crescent (mean±s.d. from three different experiments; n >30 per experiment). Spindle angles were measured between the white lines in ( d ). ( f ) Quantification of spindle misorientation towards the centre of the cortical LGN crescent (populations between 30° and 90° degrees in ( e ). ( g ) The x – z projections of metaphase cells transfected with ABL1 siRNA together with GFP alone, GFP-FL-NuMA-YE or GFP-FL-NuMA-YF, and stained with anti-LGN and anti-γ-tubulin antibodies and Hoechst (blue). The signals for LGN and γ-tubulin are shown in green and red, respectively. GFP signals are not shown. ( h ) Distribution (histogram; n =30) and the average (inset; mean±s.e.m. from four different experiments; n =30 per experiment) of spindle angles about the z axis in the cells transfected with the indicated siRNAs together with the indicated plasmids. * P <0.05, analysed by t -test (right). Scale bars, 5 μm. Full size image For more than a quarter of a century, since the asymmetric cell division was reported in Caenorhabditis elegans and Drosophila , a genome-wide survey to identify the genes required for spindle orientation has been performed exclusively in the invertebrate model organisms. Here we establish a new high-throughput screen method to survey the genes required for spindle orientation in mammalian cells and identify ABL1 as a novel regulator for this mechanism in both culture cells and mouse epidermis. Additional candidate genes reported herein ( Supplementary Table S1 ) suggest that a number of previously unrecognized kinases are involved in regulating spindle orientation in mammals. Further studies on functions of these kinases, together with the analysis in mice in vivo , may ultimately unveil the signalling networks for the spindle orientation in mammals. ABL1 regulates cortical localization of LGN both in HeLa cells and epidermis ( Figs 2 and 3 ). Although recent studies show that ABL1 regulates cadherin-dependent cell adhesions [33] and that spindles are misoriented in the α-catenin-null epidermis [9] , it seems unlikely that a defect in adherens junctions is a cause of the LGN mislocalization and spindle misorientation in the ABL1-deficient cells because LGN is no longer localized to the cortex in α-catenin-null epidermis [9] , whereas it still forms a crescent at the cortex in ABL1 KO epidermis ( Fig. 3d and e ). In addition, cell-cell adhesion is not involved in the spindle orientation control in HeLa cells [6] . It is reported that, in Drosophila neuroblasts, the Dlg-mediated attachment of astral microtubules to the cortex induces the cortical Pins polarity in the absence of functional Par proteins [19] . As HeLa cells lack cell polarity, it would be possible that ABL1 regulates cortical localization of LGN through the astral microtubules/Dlg pathway. We show that ABL1 directly phosphorylates NuMA on Tyr 1774 ( Fig. 4 ). This phosphorylation is dispensable for the association between NuMA and LGN or the NuMA-dependent cortical recruitment of LGN ( Fig. 4e ; Supplementary Fig. S13 and S14 ), but is required for anchoring NuMA at the cortex during metaphase to orient the spindle towards LGN crescent ( Fig. 5 ). As the microtubule binding domain of NuMA overlaps with the LGN binding domain, NuMA cannot binds astral microtubules at the same time as it binds LGN [32] . Thus, it is believed that NuMA is released from the LGN–Gα complex and anchored to the cortex during metaphase by unknown mechanisms before it associates with astral microtubules at the cortex [16] , [32] . Our results thus identify, for the first time, ABL1 as a key molecule in this anchoring mechanism. Importantly, the replacement of endogenous NuMA by NuMA-YF does not induce the cortical accumulation of LGN, which was induced by the ABL1 depletion ( Fig. 4e ). Therefore, ABL1 would suppress the cortical accumulation of LGN through other target molecule(s) that is distinct from NuMA. We demonstrate that ABL1 regulates spindle orientation by two mechanisms. It suppresses the cortical accumulation of LGN to prevent the LGN/Dlg-induced abnormal rotation of the spindle, and it directly phosphorylates NuMA on Tyr 1774, which is required for its anchoring at the cortex to orient spindles towards the LGN crescent ( Fig. 6 ). 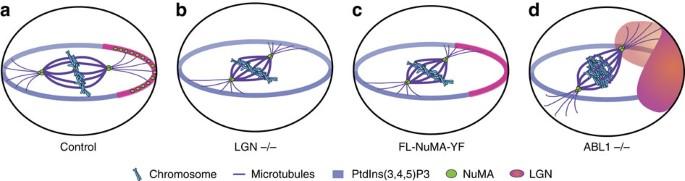Figure 6: A model for the ABL1-mediated spindle orientation control. (a) Under normal condition, ABL1 regulates spindle orientation by two mechanisms: (1) suppresses the accumulation of LGN at the cortex to prevent the LGN/Dlg-induced abnormal spindle rotation along thezaxis. This ensures the PI(3)K–PtdIns(3,4,5)P3 pathway functions normally to orient the spindle parallel to the substratum and (2) directly phosphorylates NuMA on Tyr 1774 to sustain the cortical localization of NuMA during metaphase, which is required for the spindle orientation towards the LGN crescent on thex–yplane. (b) In the absence of LGN, NuMA fails to localize at the cortex, but spindles are properly orientated about thezaxis by the PI(3)K–PtdIns(3,4,5)P3-dependent mechanism. (c) When the endogenous NuMA is replaced by NuMA Y1774F, spindles are properly oriented about thezaxis, probably by the PI(3)K–PtdIns(3,4,5)P3-dependent mechanism, but fails to align towards the LGN crescent on thex–y plane due to the absence of NuMA at the cortex. (d) In the ABL1-depleted cells, NuMA fails to localize at the cortex, whereas LGN is broadly localized at the cortex along thezaxis, which results in the LGN/Dlg-dependent abnormal rotation of the spindle and thus spindle misorientation about thezaxis. We show only LGN crescent at one pole, even though it is present at both poles in a significant population of HeLa cells. Figure 6: A model for the ABL1-mediated spindle orientation control. ( a ) Under normal condition, ABL1 regulates spindle orientation by two mechanisms: (1) suppresses the accumulation of LGN at the cortex to prevent the LGN/Dlg-induced abnormal spindle rotation along the z axis. This ensures the PI(3)K–PtdIns(3,4,5)P3 pathway functions normally to orient the spindle parallel to the substratum and (2) directly phosphorylates NuMA on Tyr 1774 to sustain the cortical localization of NuMA during metaphase, which is required for the spindle orientation towards the LGN crescent on the x – y plane. ( b ) In the absence of LGN, NuMA fails to localize at the cortex, but spindles are properly orientated about the z axis by the PI(3)K–PtdIns(3,4,5)P3-dependent mechanism. ( c ) When the endogenous NuMA is replaced by NuMA Y1774F, spindles are properly oriented about the z axis, probably by the PI(3)K–PtdIns(3,4,5)P3-dependent mechanism, but fails to align towards the LGN crescent on the x –y plane due to the absence of NuMA at the cortex. ( d ) In the ABL1-depleted cells, NuMA fails to localize at the cortex, whereas LGN is broadly localized at the cortex along the z axis, which results in the LGN/Dlg-dependent abnormal rotation of the spindle and thus spindle misorientation about the z axis. We show only LGN crescent at one pole, even though it is present at both poles in a significant population of HeLa cells. Full size image ABL1 KO mice have defects in lymphocyte development [13] , [14] , and BCR-ABL1 causes chronic myeloid leukaemia. Given the growing evidence for the implication of spindle misorientation with tumour development [3] , [4] , it is important to examine the possible role of the ABL1-mediated spindle orientation control in the lymphocyte development and its oncogenic function in chronic myeloid leukaemia. Spindle orientation has an essential role in morphogenesis, asymmetric cell division and stem cell self-renewal. Our findings should contribute to the elucidation of the mechanisms underlying these phenomena. Cell culture and antibodies HeLa cells and HeLa cells stably expressing GFP-H2B (HeLa-GH2B) were cultured in Dulbecco's Modified Eagle's Medium with 10% fetal bovine serum. In all experiments, cells were cultured on fibronectin and synchronized by a double-thymidine block. Imatinib methanesulfonate (Gleevec; Novartis) was dissolved in water (2 mM) and stored at −20 °C. The antibodies used included anti-ABL1 (Calbiochem and Santa Cruz), anti-CrkL (Santa Cruz), anti-p-CrkL (Cell Signaling), anti-GFP (Clontech), anti-α-tubulin (Sigma), CY3-conjugated anti-β-tubulin (Sigma), anti-γ-tubulin (Sigma), anti-SAP97 (hDlg; Santa Cruz), anti-NuMA (Santa Cruz and Calbiochem), anti-LGN (F Matsuzaki), anti-Dvl1 (Santa Cruz), anti-Dvl2 (Cell Signaling), anti-Dvl3 (Santa Cruz), anti-β4 integrin (BD Pharmingen), anti-β1 integrin (Chemicon), anti-PAK2 (Upstate) and anti-myc (Santa Cruz). Spindle-orientation analysis Z-stack images (0.5 μm apart) of metaphase cells stained with anti-γ-tubulin and anti-α-tubulin antibodies and Hoechst were obtained, and were subjected to our homemade ImageJ plugin. This plugin defines the position of the two poles of a spindle in a series of the Z-stack images, and measures the linear distance and the vertical distance between the two poles of a metaphase spindle, and calculates the spindle angle by inverse trigonometric function. Cell preparation for an RNAi screen For the first screening, HeLa-GH2B cells were transfected with each siRNA (6 pmol) of a Silencer Kinase siRNA library (targeting 719 genes, three kinds of siRNAs/gene, 2,157 siRNAs in total; Ambion) by using siPort Neo Fx (Ambion) in the 96-well tissue culture plates (BD Bioscience), which were pre-coated with fibronectin, and synchronized by a double-thymidine block. Ten hours after the release from a double-thymidine block, when the majority of the cells entered mitosis, cells were fixed and stained with anti-CY3-conjugated–anti-β-tubulin antibody and Hoechst. For the second screening, HeLa cells were cultured in the fibronectin-coated 96-well tissue culture plates, transfected with each siRNA (10 pmol) by using Oligofectamine, incubated for 4 h and synchronized by a double-thymidine block. Ten hours after release from a double-thymidine block, cells were fixed and stained with anti-γ-tubulin and anti-α-tubulin antibodies and Hoechst, then subjected to the spindle-orientation analysis. siRNA experiments The siRNAs of human LGN, Dlg1, Dvl1, Dvl2 and Dvl3 were designed targeting on the sequence as follows: LGN, 5′-gctgcagttcaagttggaact-3′; Dgl1, 5′-gctctactgtgacttcaga-3′; Dvl1, 5′-ggaggagatctttgatgac-3′; Dvl2, 5′-ggaagaaatttcagatgac-3′; Dvl3, 5′-ggaggagatctcggatgac-3′ [22] , [26] , [34] . The siRNA of human NuMA was designed targeting on the sequence as follows: 5′-ggcgaggcaggagaagaac-3′. Oligonucleotides were purchased from Japan Bioservice. The siRNAs of human ABL1 were purchased from Ambion (ABL1-1si:Ambion siRNA ID 1336; ABL1-2si:Ambion siRNA ID 1431). HeLa cells were transfected with siRNA by using Oligofectamine (Invitrogen), incubated for 4 h and synchronized by a double-thymidine block. The expression levels of the proteins were analysed by western blot. Plasmid constructs and transfection FL mouse ABL1 cDNA (a gift from M Matsuda) was subcloned into pCS2 and pcDNA3. GFP-mouse ABL1-wt and GFP-mouse ABL1-kd were from N Watanabe [35] . GFP-Dvl2 was from A Kikuchi [24] . NuMA-C (aa 1,700—2,116) cDNA and FL LGN cDNA were amplified with Kod plus DNA polymerase (Toyobo) by using HeLa cDNA library as a template with the following primer pairs: NuMA-C, 5′-cccctccaggaaggaacagcttctac-3′ and 5′-ccagtcatccagctgctcaggct-3′; LGN, 5′-gcctcgagctatggaggaaaatttgataagcatgagagaagacc-3′ and 5′-ccgtcgacctaatggtctgccg-3′. The amplified products were subcloned into pGEX-6P1 and pEGFP-C (Clontech), respectively. FL NuMA cDNA was obtained by amplifying and conjugating the DNA segments by using the following primer pairs: 5′-atagatctatgacactccacgccacccgg-3′ and 5′-gcttcaaggtctcgagctgcaagacatcac-3′; 5′-gtgatgtcttgcagctcgagaccttgaagc-3′ and 5′-gcagggtagcgaattccacacgctgc-3′; 5′-gcagcgtgtggaattcgctaccctgc-3′ and 5′-gggcagtcgactgtgcttctcgctg-3′; 5′-cagcgagaagcacagtcgactgccc-3′ and 5′-tccagggacgctggtaccgtctgg-3′; 5′-ccagacggtaccagcgtccctgga-3′ and 5′-ccggatccttagtgctttgccttgccc-3. NuMA-YE, NuMA-YF and Dvl2-YF were constructed by mutagenesis using QuickChange Site-Directed Mutagenesis Kit (Stratagene). HeLa cells were transfected with plasmids by using Lipofectamine Plus (Invitrogen) after the first release of a double-thymidine block, incubated for 1 h and washed with the fresh medium. Time-lapse imaging and spindle-rotation analysis HeLa cells were transfected with siRNAs by using Oligofectamine (Invitrogen), incubated for 4 h and subjected to a double-thymidine block. At the time of secondary thymidine treatment, cells were trypsinized and plated onto Lab-Tek 8-well chambered coverglass (Nunc), incubated for 15 h to be synchronized in G1/S phase. Ten hours after release from a double-thymidine block, cells were treated with MG132 for 30 min to be arrested in metaphase. Before acquisition, cells were pre-incubated with Hoechst to label the chromosomes. During acquisition, cells were cultured in the medium with 20 mM HEPES (pH 7.3). Time-lapse images were obtained by Olympus IX81-ZDC microscope with a temperature-controlled and motorized stage and by Meta Morph software. Time-lapse images were taken every 5 min for 90 min. The acquired images of Hoechst at each time point were binarized to white and black by using Meta Morph software. The white area represents the chromosome, and white pixels were measured as relative chromosome area. We judged that the chromosomes were tilted along the z axis when the relative chromosome area exceeded 1.5. Supplementary Fig. S17 shows the relative chromosome area in each time point obtained from the time-lapse images of Supplementary Movie 4 , 5 and 6 . Immunoprecipitations For immunoprecipitation of PAK2, M-phase-synchronized HeLa cells were washed with PBS and lysed in buffer A (50 mM Hepes (pH 7.4), 10 mM 2-glycerophosphate, 50 mM NaCl, 2 mM MgCl 2 , 2 mM EGTA, 1 mM EDTA, 15 mM NaF, 10% glycerol, 0.5% NP-40, 5 mM dithiothreitol, 1 mM phenylmethylsulfonyl fluoride, 5 mM Na 3 VO 4 , and 2 μg ml −1 aprotinin). The cell lysates were centrifuged at 20,000 g for 15 min and the supernatants (cell extracts) were incubated with anti-PAK2 antibody or rabbit IgG coupled to the Protein A-Sepharose (Pharmacia Corp.) for 3 h [8] . For immunoprecipitation of Myc-tagged NuMA, cells were transfected with plasmids encoding myc-FL-NuMA, myc-C-NuMA or the empty vector after the first release from a double-thymidine block, incubated for 1 h and washed with the fresh medium. Ten hours after release of a double-thymidine block, cell extracts were prepared and incubated with anti-myc antibody coupled to the Protein A-Sepharose for 3 h. The bead complexes were washed three times with buffer A and subjected to immunoblotting. Protein preparation and kinase assays The recombinant proteins of GST-NuMA-C-wt and GST-NuMA-C-YF were expressed in Escherichia coli and purified by affinity chromatography on glutathione-Sepharose 4B (GE Healthcare). The recombinant protein of GST-ABL1 kinase domain was purchased from Cell Signaling. GST-ABL1 kinase domain was mixed with GST-NuMA-C-wt, GST-NuMA-C-YF or GST-Crk (Upstate), together with 50 μM ATP, and 15 mM MgCl 2 in a final volume of 15 μl, and then incubated for 10, 20, 30 s, 1, 5 or 10 min at 30 °C in the presence of 3 μCi of [γ- 32 P] ATP. The reactions were stopped by the adding Laemli's sample buffer and by boiling. Cell staining For detecting LGN, hDlg1 and NuMA, cells were fixed with 10% trichloroacetic acid followed by incubation with methanol at −20 °C for 10 min. For detection of α-tubulin and γ-tubulin, cells were fixed with 3.7% formaldehyde at 37 °C for 5 min, followed by incubation with methanol at −20 °C for 20 min. Cells were blocked with 3% BSA at 37 °C for 30 min, incubated with primary antibodies at 4 °C overnight, washed and incubated for 1 h with secondary antibodies (AlexaFluor 488- or 594-goat anti-mouse, anti-rabbit or anti-rat IgG antibodies (Molecular Probes)). Mouse preparation and histological analysis We performed all animal experiments in accordance with the Regulation on Animal Experimentation at Kyoto University. For imatinib treatment, C57BL/6 mice received intraperitoneal injections of imatinib mesylate (Gleevec) (4 mg kg −1 ) twice at 12-h intervals. C57BL/6 mice carrying a heterozygous mutation in the ABL1 gene were kindly donated by RC Mulligan [14] . ABL1 genotyping was performed by PCR using the following primer pairs: abl1 , 5′-atggaggtggaggagttcctga-3′ and 5′-aatggtggttcccgggtacaca-3′; neo , 5′-ggagaggctattcggctatgac-3′ and 5′-cgcattgcatcagccatgatgg-3′ (ref. 14 ). For detection of LGN, NuMA and β4-integrin, embryos were fixed with 10% trichloroacetic acid. For detection of ABL1 and β1-integrin, embryos were fixed with 4% paraformaldehyde, cryoprotected in PBS/20% sucrose and frozen in Optimal Cutting Temperature compound. The fixed embryos were cut into slices and subjected to immunostaining. For detection of NuMA at the cell cortex, after cryosection, samples were permeabilized with 0.5% Triton-X100 in TE buffer (10 mM Tris-HCl (pH 9.0) and 1 mM EDTA) for 30 min at 37 °C. How to cite this article: Matsumura, S. et al . ABL1 regulates spindle orientation in adherent cells and mammalian skin. Nat. Commun. 3:626 doi: 10.1038/ncomms1634 (2012).